Molecular basis for class Ib anti-arrhythmic inhibition of cardiac sodium channels Cardiac sodium channels are established therapeutic targets for the management of inherited and acquired arrhythmias by class I anti-arrhythmic drugs (AADs). These drugs share a common target receptor bearing two highly conserved aromatic side chains, and are subdivided by the Vaughan-Williams classification system into classes Ia-c based on their distinct effects on the electrocardiogram. How can these drugs elicit distinct effects on the cardiac action potential by binding to a common receptor? Here we use fluorinated phenylalanine derivatives to test whether the electronegative surface potential of aromatic side chains contributes to inhibition by six class I AADs. Surprisingly, we find that class Ib AADs bind via a strong electrostatic cation–pi interaction, whereas class Ia and Ic AADs rely significantly less on this interaction. Our data shed new light on drug-target interactions underlying the inhibition of cardiac sodium channels by clinically relevant drugs and provide information for the directed design of AADs. Voltage-gated sodium channels contribute to the cadence and membrane stability in the heart by driving the upstroke of the cardiac action potential. These large (~220 kD) membrane proteins consist of four homologous domains (DI-DIV), each containing six transmembrane alpha-helical segments (S1–S6). The S1–S4 segments house a voltage-sensing domain that is tightly coupled to the S5-pore helix-S6 segments that form the selectivity filter and permeation pathway [1] . Nine sodium channel proteins (Na V 1.1–Na V 1.9) show distinct physiology and expression in the excitable cells of the cardiovascular and nervous systems [2] , with Na v 1.5 being the predominant isoform in the heart [3] . Inherited or acquired sodium channel dysfunction resulting in excessive sodium conductance can lead to cardiac arrhythmia [4] , epilepsy [5] , and enhanced pain syndromes [6] . Therapeutics that inhibit sodium conductance are widely employed to subdue the excessive membrane excitability associated with these diseases. One such family of compounds, the Vaughan–Williams class Ia–c anti-arrhythmics are valuable tools for the management of cardiac arrhythmias owing to their potent use-dependent inhibition of sodium channels [7] . This trait is due to a drug-binding preference for open and inactivated channels, two states that become dominant during the prolonged depolarizations and high firing rates that typify cardiac arrhythmias. However, the categorization of class Ia-c drugs is currently based on how they affect electrocardiographic rhythms, and not mechanistically on their molecular interactions with sodium channels, largely because this valuable information remains unknown. Class Ia drugs increase action potential duration (APD) and exhibit a moderate reduction of the phase 0 slope (for example, cause a slowing of the initial depolarization) and an increase in the effective refractory period (ERP); class Ib drugs reduce APD and show only a small decrease in the phase 0 slope and decrease the ERP, whereas class Ic drugs have no effect on APD and ERP but produce a pronounced decrease in the slope of phase 0 (refs 8 , 9 ). In practice, the use of class I therapeutics can be associated with critical contraindications for different types of atrial and ventricular arrhythmias. For instance, although some class Ic compounds are effective in managing atrial arrhythmias, the CAST (cardiac arrhythmia suppression trial) demonstrated that the use of the class Ic drugs flecainide or encainide in cases of arrhythmia, associated with structural heart disease, can lead to sudden cardiac death [10] , [11] . Flecainide is still used in clinical settings when no contraindications are present, yet the structurally similar drug encainide has been withdrawn from clinical use because of its pro-arrhythmic properties. This example highlights the need for a better molecular understanding of the characteristics that distinguish potentially harmful channel inhibitors from those with more benign profiles. It is generally appreciated that sodium channel inhibitor action involves a number of different mechanisms [12] including pore block [13] , electrostatic interactions between the cationic charge on the drug and sodium ions at the selectivity filter [14] , [15] , stabilization of either fast or slow non-conducting states of the channel [16] , [17] , gating charge immobilization [18] , [19] , [20] , and targeted uncoupling of channel gating from voltage-sensing [21] . Previous studies have shown that site-directed mutation of two strictly conserved aromatic residues in transmembrane segment 6 (S6) of the fourth sodium channel domain (DIV), Phe1760 and Tyr1767 in Na v 1.5, can virtually abolish channel inhibition by all classes of anti-arrhythmic drugs [12] , [22] , [23] , [24] . A recent study using unnatural amino-acid derivatives of aromatic phenylalanine side chains has demonstrated that skeletal sodium channels form a cation–pi interaction with lidocaine and QX-314 at aromatic residue Phe1579 (Phe1760 in Na V 1.5), but not Tyr1586 (Tyr1767 in Na V 1.5) [25] . This class of electrostatic interaction occurs between a cation and the negative potential formed by the quadrupole moment on the face of an aromatic side chain [26] , [27] and has been shown to be responsible for ligand-receptor interactions in a variety of ion channels [28] , [29] , [30] . However, it remains to be shown whether such a cation–pi interaction is conserved in the cardiac sodium channel isoform and, more importantly, whether it is a general trait of all class I anti-arrhythmic drugs. Such information would be crucial for the rational design of the next generation of safer and more specific sodium channel therapeutics. Here we set out to investigate whether the existence of a cation–pi interaction with either of two conserved aromatic side chains in the sodium channel drug receptor could be predictive in determining class I a-c anti-arrhythmic drugs. Our results demonstrate that class Ib anti-arrythmic drugs bind via a strong electrostatic cation–pi interaction to Phe1760, whereas class Ia and Ic anti-arrythmic drugs rely significantly less on the electronegative surface potential of this side chain. We conclude that a strong cation–pi interaction with Phe1760 serves as the molecular basis for the inhibition of cardiac sodium channels by class Ib anti-arrythmic drugs. 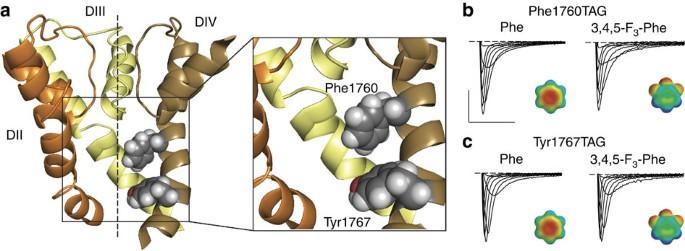Figure 1: A sodium channel homology model andin vivononsense suppression in the cardiac sodium channel. (a) Sodium channel homology model showing the S6 segments, the selectivity filter and pore helix of DII to DIV. In the left hand panel, the dashed line indicates the predicted ion permeation pathway, the right-hand panel is a magnified view of the two aromatics studied here, Phe1760 and Tyr1767. (b)/(c) Series of inward currents induced by voltage steps from −50 to +10 mV (10 mV increments) after co-injection of Nav1.5 Phe1760TAG (b) or Tyr1767TAG (c) mRNA and tRNAs coupled to Phe or 3,4,5-F3-Phe. Insets show electrostatic potential maps of the incorporated amino acid where red and blue correspond to negative (−20 kcal mol−1) and positive (+20 kcal mol−1), respectively. Note that, here, and in all following figures, the dashed lines indicate the zero-current level; the vertical and horizontal scale bars represent 1.0 μA and 5.0 ms, respectively. Incorporation of unnatural amino acids in Na V 1.5 Figure 1a shows a homology model of the cardiac sodium channel Na V 1.5 pore domain based on the structure of the voltage-gated Shaker family potassium channel K V 1.2–2.1 paddle chimera (PDB 2R9R ). The model suggests that the two aromatic side chains of residues Phe1760 and Tyr1767 reside approximately two turns apart within an α-helical section of S6 in domain IV, just below the putative selectivity filter. Importantly, their side chains are orientated towards the permeation pathway, where they could possibly interact with sodium channel inhibitors. In vivo nonsense suppression was used to incorporate serially fluorinated phenylalanine derivatives at either Phe1760 or Tyr1767 ( Fig. 1b/c ), which produced robust sodium currents with normal voltage-dependence of gating ( Supplementary Fig. S1 and Table 1 ). Such unnatural side chains are valuable research tools for studies of this type because they provide a hypothesis to be tested when investigating cation–pi interactions: each fluorine atom serially diminishes the binding energy of the putative cation–pi interaction [26] , [27] , [31] . Figure 1: A sodium channel homology model and in vivo nonsense suppression in the cardiac sodium channel. ( a ) Sodium channel homology model showing the S6 segments, the selectivity filter and pore helix of DII to DIV. In the left hand panel, the dashed line indicates the predicted ion permeation pathway, the right-hand panel is a magnified view of the two aromatics studied here, Phe1760 and Tyr1767. ( b )/( c ) Series of inward currents induced by voltage steps from −50 to +10 mV (10 mV increments) after co-injection of Na v 1.5 Phe1760TAG ( b ) or Tyr1767TAG ( c ) mRNA and tRNAs coupled to Phe or 3,4,5-F 3 -Phe. Insets show electrostatic potential maps of the incorporated amino acid where red and blue correspond to negative (−20 kcal mol −1 ) and positive (+20 kcal mol −1 ), respectively. Note that, here, and in all following figures, the dashed lines indicate the zero-current level; the vertical and horizontal scale bars represent 1.0 μA and 5.0 ms, respectively. Full size image Table 1 Conductance-voltage and steady-state inactivation data. Full size table Conserved charge distribution in anti-arrhythmic drugs Previous studies have established that cationic charge is an important determinant of local anaesthetic and anti-arrhythmic use-dependent inhibitory potency [25] , [32] , [33] , [34] . To explore this property further, we employed ab initio predictions of structure and electrostatic potential to better resolve the subtle nuances in drug shape and distribution of cationic charge. 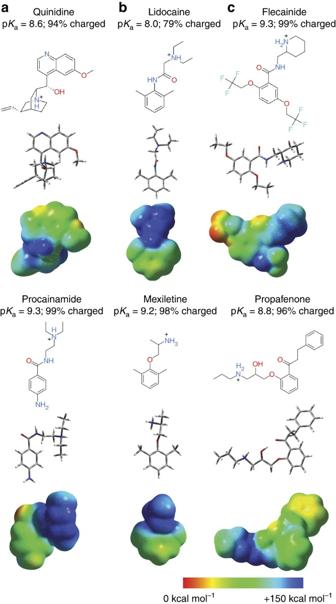Figure 2:Ab Initiocalculations predict the electrostatic potential distributions of anti-arrhythmic drugs. All class I anti-arrhythmic drugs tested here are displayed as chemical structures (upper panels), energy-minimized three-dimensional structures (equatorial panels), and electrostatic potential maps (lower panels). (a) to (c) Class Ia, Ib and Ic anti-arrhythmic drugs, respectively. pKavalues and the predicted percentage of protonated drug at pH 7.4 are indicated. The scale bar indicates electrostatic surface potentials from 0 kcal mol−1(red) to +150 kcal mol−1(blue). The results of this analysis are shown in Figure 2 , where the protonated species of the drugs (upper panels), energy-minimized structures (middle panels), and energy-minimized structures with the predicted electrostatic surface potentials are compared (bottom panels). The drugs tested here are protonated to variable degrees at pH 7.4 ( Table 2 ) and our results suggest that at physiological pH all class I drugs show the positive electrostatic potential densities that would allow for a cation–pi interaction with aromatic side chains in the sodium channel drug receptor. Figure 2: Ab Initio calculations predict the electrostatic potential distributions of anti-arrhythmic drugs. All class I anti-arrhythmic drugs tested here are displayed as chemical structures (upper panels), energy-minimized three-dimensional structures (equatorial panels), and electrostatic potential maps (lower panels). ( a ) to ( c ) Class Ia, Ib and Ic anti-arrhythmic drugs, respectively. p K a values and the predicted percentage of protonated drug at pH 7.4 are indicated. The scale bar indicates electrostatic surface potentials from 0 kcal mol −1 (red) to +150 kcal mol −1 (blue). Full size image Table 2 Physicochemical properties of the drugs tested. 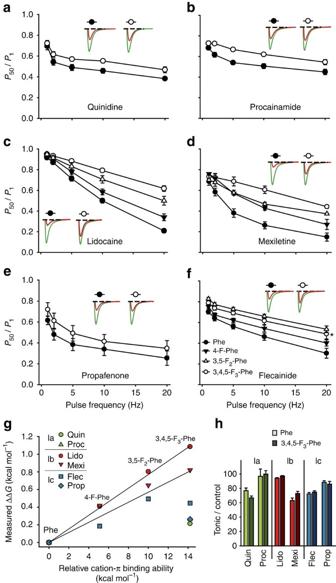Figure 3: A strong cation–pi interaction for class Ib anti-arrhythmic drugs under use-dependent, but not tonic conditions. (a–f) Fractional-current level remaining after the 50th pulse (P50/P1) as a function of the pulse rate with different unnatural amino acids incorporated at position 1760 in the presence of class Ia 100 μM quinidine (a) and 10 mM procainamide (b); class Ib 50 μM lidocaine (c) and 100 μM mexiletine (d) and class Ic 25 μM propafenone (e) and 20 μM flecainide (f). The insets compare the control current level (green) with the current level after the 50th pulse (red) at 20 Hz. Note that although a 20 Hz stimulation is likely a faster stimulation than one would expect even under pathological conditions, this protocol serves to highlight the use-dependence of drug binding. Also note that 4-F-Phe and 3,5-F2-Phe were only employed for lidocaine, mexiletine and flecainide (see text). The asterisk in (f) indicates the inhibition with 3,4,5-F3-Phe in the presence of flecainide. (g) Cation–pi plot for class I anti-arrythmic drugs. Class Ia data Quin and Proc) are shown in green, class Ib data (Lido and Mexi) are shown in red, class Ic data (Flec and Prop) are shown in blue. Inhibitory constants were estimated as described25and the approach was validated with full concentration-response curves for quinidine, lidocaine and propafenone (Supplementary Fig. S2). Briefly, 20 Hz data were used to calculate the energetic effect of fluorination at Phe1760 (ΔΔG). Binding energy is defined as 0.58ln(Ki,mut/Ki,wt) kcal/mol, whereKi,mut/Ki,wt is the fractional increase in the inhibitory constant caused by an unnatural mutant compared with benzene/phenylalanine. The relative cation–pi binding ability plotted on the X-axis is derived from calculations that predict the interaction energetics of a sodium ion with benzene30. A y0=0 constraint was used for the linear fits for better comparison. (h) Bar diagram comparing tonic (0.2 Hz) inhibition of all drugs tested here with Phe (light-coloured bars) or 3,4,5-F3-Phe (dark-coloured bars) incorporated at position 1760; colour-coding as in (g). Data shown as mean+s.e.m. (n=4–11). Flec, flecainide; Lido, lidocaine; Mexi, mexiletine; Proc, procainamide; Prop, propafenone; Quin, quinidine. Full size table A strong cation–pi interaction for class Ib drugs Figure 3 shows the effects of serial fluorination of Phe1760 on use-dependent channel inhibition by class Ia anti-arrhythmic drugs. Representative current traces ( Fig. 3a ) are shown in the presence of quinidine before (green) and after (red) 50 consecutive steps from −100 mV to −20 mV at a pulse rate of 20 Hz for channels containing Phe and 3,4,5-F 3 -Phe at position 1760, respectively. In this case, Phe and 3,4,5-F 3 -Phe, shown in open and closed circles, respectively, were similarly inhibited ( P =0.03), indicating that the inhibition by quinidine is not mediated by a strong cation–pi interaction (although a weak contribution of the electronegative surface potential of Phe1760 to quinidine is likely). Although the single 3,4,5-F 3 -Phe substitution cannot alone demonstrate a cation–pi interaction, this manipulation will drastically reduce the negative potential on the face of the side chain and would be expected to cause a substantial change in the interaction affinity, if an electrostatic interaction represents a significant portion of the interaction energy. Previously, we have shown that lidocaine forms a cation–pi interaction with the residue homologous to Phe1760 in skeletal sodium channels (Phe1579) (ref. 25 ), and, as shown in Figure 2 , the class Ia drug procainamide is very similar in structure and p K a to lidocaine, suggesting that the two compounds could have a similar cation–pi interaction in the local anaesthetic receptor. Surprisingly, trifluorination here produced only modest relief (Phe and 3,4,5-F 3 -Phe were inhibited similarly; P =0.04), arguing against a substantial contribution of the electronegative surface potential at Phe1760 in procainamide inhibition. Given the chemical and structural similarity of lidocaine and procainamide, this result raised the possibility that cardiac sodium channels show differential interactions with anti-arrhythmic drugs when compared with skeletal muscle sodium channels. However, Figure 3c shows that inhibition of cardiac channels by lidocaine is dramatically reduced with trifluorination compared with Phe at the same position (P 1 /P 50 20.8±1.9 for Phe versus 61.8±2.8 for 3,4,5-F 3 -Phe, for 7 and 10 cells, respectively, P <0.001), suggesting that the cation–pi interaction for lidocaine is conserved between skeletal and cardiac isoforms. This possibility was further confirmed by employing the mono- and di-fluoro Phe derivatives, also shown in Figure 3c . Very similar results were obtained for the class Ib drug, mexiletine ( Fig. 3d ), where each added fluorine at Phe1760 produces a linear, stepwise relief of inhibition at 20 Hz ( P 1 / P 50 14.8±3.9 for Phe versus 43.2±1.7 for 3,4,5-F 3 -Phe, for 6 cells each, P <0.001). In both examples, the class Ib compounds, lidocaine and mexiletine, rely heavily on cation–pi interactions at Phe1760, as trifluorination causes a highly significant loss in binding energy, suggesting that this contribution is a significant energetic factor in the use-dependent inhibition by class Ib drugs. Next, Figure 3e shows potent use-dependent inhibition by the class Ic anti-arrhythmic propafenone that is almost unperturbed by the 3,4,5-F 3 -Phe derivative over a wide range of pulse frequencies ( P =0.05). In Figure 3f, we tested the class Ic drug flecainide, where interestingly, the 3,4,5-F 3 -Phe produced some relief when compared with Phe ( P =0.02), prompting us to explore the interaction in more detail with the mono- and di-fluoro Phe derivatives. However, the 3,4,5-F 3 -Phe caused less disruption than 3,5-F 2 -Phe, a result that is inconsistent with a cation–pi interaction, thereby ruling out the possibility of a strong cation–pi interaction between Phe1760 and flecainide. However, a small contribution of the electronegative surface potential of Phe1760 to flecainide inhibition remains a possibility. Figure 3: A strong cation–pi interaction for class Ib anti-arrhythmic drugs under use-dependent, but not tonic conditions. ( a–f ) Fractional-current level remaining after the 50th pulse (P 50 /P 1 ) as a function of the pulse rate with different unnatural amino acids incorporated at position 1760 in the presence of class Ia 100 μM quinidine ( a ) and 10 mM procainamide ( b ); class Ib 50 μM lidocaine ( c ) and 100 μM mexiletine ( d ) and class Ic 25 μM propafenone ( e ) and 20 μM flecainide ( f ). The insets compare the control current level (green) with the current level after the 50th pulse (red) at 20 Hz. Note that although a 20 Hz stimulation is likely a faster stimulation than one would expect even under pathological conditions, this protocol serves to highlight the use-dependence of drug binding. Also note that 4-F-Phe and 3,5-F 2 -Phe were only employed for lidocaine, mexiletine and flecainide (see text). The asterisk in ( f ) indicates the inhibition with 3,4,5-F 3 -Phe in the presence of flecainide. ( g ) Cation–pi plot for class I anti-arrythmic drugs. Class Ia data Quin and Proc) are shown in green, class Ib data (Lido and Mexi) are shown in red, class Ic data (Flec and Prop) are shown in blue. Inhibitory constants were estimated as described [25] and the approach was validated with full concentration-response curves for quinidine, lidocaine and propafenone ( Supplementary Fig. S2 ). Briefly, 20 Hz data were used to calculate the energetic effect of fluorination at Phe1760 (ΔΔG). Binding energy is defined as 0.58ln( K i,mut/ K i,wt) kcal/mol, where K i,mut/ K i,wt is the fractional increase in the inhibitory constant caused by an unnatural mutant compared with benzene/phenylalanine. The relative cation–pi binding ability plotted on the X-axis is derived from calculations that predict the interaction energetics of a sodium ion with benzene [30] . A y0=0 constraint was used for the linear fits for better comparison. ( h ) Bar diagram comparing tonic (0.2 Hz) inhibition of all drugs tested here with Phe (light-coloured bars) or 3,4,5-F 3 -Phe (dark-coloured bars) incorporated at position 1760; colour-coding as in ( g ). Data shown as mean+s.e.m. ( n =4–11). Flec, flecainide; Lido, lidocaine; Mexi, mexiletine; Proc, procainamide; Prop, propafenone; Quin, quinidine. Full size image Formalizing the cation–pi interaction for class Ib drugs An advantage of the approach used here over traditional site-directed mutagenesis is that for a true cation–pi interaction, serial fluorination will produce a stepwise reduction in binding energy with each added fluorine atom. We calculated an approximate binding affinity (at 20 Hz) for the drugs tested and the change in binding energy (ΔΔ G ) that was measured from channels with fluorination plotted against the ab initio -calculated relative cation–pi binding energy ( Fig. 3 ). As shown in Figure 3g , a clear linear relation between binding affinity and cation–pi binding ability is observed for lidocaine and mexiletine, demonstrating that these class Ib anti-arrhythmic drugs form a strong cation–pi interaction with Phe1760. In this case, the abscissa is derived from ab initio gas phase calculations that demonstrate the predicted stepwise loss in binding energy between an idealized cation, sodium, and a benzene ring with one, two or three appended fluorine atoms [31] . Whereas this system serves as a rough approximation for the diffuse quaternary ammonium moiety of the compounds studied here, the linear trend is valid for the identification of any cation–pi interaction. Moreover, this approach is helpful, because it allows for the straightforward comparison of the present study with other previously characterized cation–pi systems through the relative slope of the plot. For instance, viewing our results in light of previously confirmed cation–pi interactions in ligand-gated channels where, although the drug/receptor ratio is different (1:1 for anti-arrhythmic drugs and sodium channels; at least 2:1 for pentameric ligand-gated channels and their agonists), the slopes of the cation–pi plots for lidocaine and mexiletine (−0.08 and −0.06, respectively) are similar to those observed for activation of the nicotinic acetylcholine receptor with acetylcholine (−0.11) [35] and the activation of the glycine receptor with β-alanine and taurine (−0.12 and −0.09, respectively) [36] . To test whether the observed trend of serial fluorination-induced relief of inhibition for class Ib drugs persisted at more physiological temperatures, we investigated the effect of fluorination on inhibition by quinidine, lidocaine and propafenone at 31 °C (temperatures of more than 32 °C resulted in unstable recording conditions). Interestingly, we found that the relative level of inhibition between Phe and 3,4,5-F 3 -Phe under use-dependent conditions was not significantly different compared with experiments performed at room temperature ( Supplementary Fig. S3 ), further underlining the relevance of this observation. No electrostatic contribution at Phe1760 in tonic blockade We also examined the contribution of Phe1760 to the inhibition of 'resting channels', shown in Figure 3h , and found no cation–pi interaction with any of the compounds tested here, when channels are depolarized infrequently (0.2 Hz). Whereas this observation provides interesting mechanistic insights (Discussion), we can also conclude that the electrostatic surface potential of Phe1760 is not crucial for tonic inhibition. Clues from class I anti-arrhythmic drug derivatives To further elucidate why lidocaine, but not the structurally similar drug procainamide, forms a strong cation–pi interaction with Phe1760, we turned to a series of anti-arrhythmic drug derivatives that have very similar structures to known class I anti-arrhythmic drugs but have not been classified within the Vaughan-Williams system. We specifically aimed to assess the effects of adding modifying groups at or near the tertiary amine group or along the edge of the aromatic benzene moiety. Supplementary Figure S4 shows the energy-minimized structures and corresponding electrostatic surface potential maps for the compounds employed in the subsequent analysis. Here, as in Figure 3 , the electrostatic surface potential maps for the compounds suggest that all possess the prerequisite cationic densities that could potentially allow them to engage in cation–pi interactions. Interestingly, adding a single methyl group to lidocaine at either the 4 position of the aromatic (methyl-4-para-lidocaine; Fig. 4b ) or the tertiary amine (RAD-241; Fig. 4c ) resulted in a weaker, but still energetically significant cation–pi interaction with Phe1760 ( Fig. 4g ). 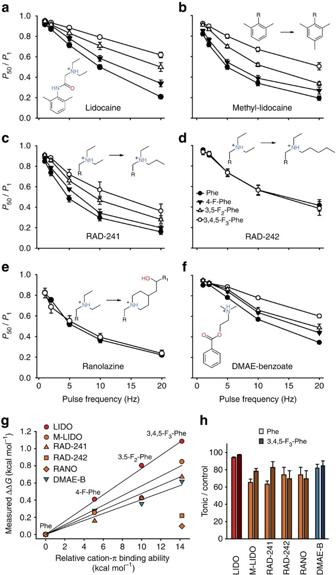Figure 4: Deciphering the molecular determinants for cation–pi interactions at Phe1760 using class I derivatives. (a–f) Fractional-current level remaining after the 50th pulse (P50/P1) as a function of the pulse rate with different unnatural amino acids incorporated at position 1760 in the presence of 50 μM lidocaine (a), 500 μM methyl-4-para-lidocaine (b), 300 μM RAD-241 (c), 250 μM RAD-242 (d), 200 μM ranolazine (e) and 500 μM 2-(dimethylamino)ethyl benzoate (DMAE-benzoate) (f). In (b–e) structural differences of the lidocaine derivatives are highlighted by the insets; R stands for the rest of the lidocaine molecule (g) Cation–pi plot for class I anti-arrythmic drug derivatives. Data for class Ib drug LIDO is shown in red, data for lidocaine derivatives M-LIDO, RAD-241 and RAD-242, as well as RANO are shown in yellow and the data for the procainamide derivative DMAE-B is shown in blue. For details about the generation of the plot seeFig. 3. (h) Bar diagram comparing tonic (0.2 Hz) inhibition of all drugs tested here with Phe (light-coloured bars) or 3,4,5-F3-Phe (dark-coloured bars) incorporated at position 1760; colour-coding as in (g). Data shown as mean+s.e.m. (n=3–8). DMAE-B, DMAE-benzoate; LIDO, lidocaine; M-LIDO, methyl lidocaine; RANO, ranolazine. However, larger alkyl or cyclic substitutions at the tertiary amine resulted in complete abolition of the cation–pi interaction (RAD-242 and ranolazine in Figure 4d, e and g ; bupivacaine in Supplementary Fig. S5 ; inhibition for Phe and 3,4,5-F 3 -Phe not significantly different at 20 Hz; P >0.2). It is important to note that ranolazine, although a direct derivative of lidocaine, no longer displays class Ib-like characteristics as it prolongs the APD and increases the ERP [37] , [38] . In contrast, we observed an energetically significant cation–pi interaction with Phe 1760 for 2-(dimethylamino)ethyl benzoate (DMAE-B) ( Fig. 4f and g ), a compound similar to procainamide, but smaller in volume and length, and free of a kinked backbone ( Supplementary Fig. S4 ). Taken together, these results suggest that the overall size of the inhibitory drugs is important to determine whether or not a drug forms an energetically significant cation–pi interaction with Phe1760. Figure 4: Deciphering the molecular determinants for cation–pi interactions at Phe1760 using class I derivatives. ( a – f ) Fractional-current level remaining after the 50th pulse (P 50 /P 1 ) as a function of the pulse rate with different unnatural amino acids incorporated at position 1760 in the presence of 50 μM lidocaine ( a ), 500 μM methyl-4-para-lidocaine ( b ), 300 μM RAD-241 ( c ), 250 μM RAD-242 ( d ), 200 μM ranolazine ( e ) and 500 μM 2-(dimethylamino)ethyl benzoate (DMAE-benzoate) ( f ). In ( b – e ) structural differences of the lidocaine derivatives are highlighted by the insets; R stands for the rest of the lidocaine molecule ( g ) Cation–pi plot for class I anti-arrythmic drug derivatives. Data for class Ib drug LIDO is shown in red, data for lidocaine derivatives M-LIDO, RAD-241 and RAD-242, as well as RANO are shown in yellow and the data for the procainamide derivative DMAE-B is shown in blue. For details about the generation of the plot see Fig. 3 . ( h ) Bar diagram comparing tonic (0.2 Hz) inhibition of all drugs tested here with Phe (light-coloured bars) or 3,4,5-F 3 -Phe (dark-coloured bars) incorporated at position 1760; colour-coding as in ( g ). Data shown as mean+s.e.m. ( n =3–8). DMAE-B, DMAE-benzoate; LIDO, lidocaine; M-LIDO, methyl lidocaine; RANO, ranolazine. Full size image The local anaesthetic benzocaine lacks an amino group that can be protonated under physiological conditions (the anilino nitrogen of benzocaine has a p K a of 2.5). Consistent with earlier studies, we found almost no use-dependent inhibition by benzocaine [20] , [25] , [33] , [39] ( Supplementary Fig. S5 ), suggesting that a protonated amine is necessary for use-dependent inhibition. However, this does not answer the question as to whether the amine of anti-arrhythmic drugs provides the positive charge in the cation–pi interaction. Although it is conceivable that the partial positive charge on the unobstructed edge of the aromatic ring of drugs such as lidocaine serves as the cation [40] , the fact that methyl-4-para-lidocaine still forms an energetically significant cation–pi interaction with Phe1760 rules out this possibility, as the added methyl group in this position of the aromatic would strongly disrupt a possible cation–pi 'edge' interaction. We conclude that the aromatic functional group is a crucial structural component of all drugs tested here, but it is unlikely to contribute to electrostatic interactions. Similar to the results shown in Figure 3h , none of the derivatives of class I anti-arrhythmic drugs tested here form a cation–pi interaction under conditions favouring tonic inhibition ( Fig. 4h ). Lack of a cation–pi interaction at Tyr1767 Phe1760 and Tyr1767 have both been shown to be important for inhibition by anti-arrhythmics [22] , and it is conceivable that class Ia and Ic drugs, while lacking a strong electrostatic interaction with Phe1760, could form such an interaction with Tyr1767. To test this possibility, we replaced Tyr1767 with Phe and 3,4,5-F 3 -Phe and as shown in Figure 1c , we observed robust inward currents that displayed virtually unchanged voltage-gating relationships for activation and inactivation ( Supplementary Fig. S1 and Table 1 ). As exemplified by the effect of mexiletine ( Fig. 5a ), the tonic inhibition was not strongly affected by substituting Tyr with Phe or 3,4,5-F 3 -Phe with any of the drugs tested here ( Fig. 5b ). Similar to previously observed results [25] , [41] , all drugs displayed reduced inhibition at a pulse rate of 20 Hz with Phe at position 1767 compared with Tyr (wild type (WT)) or 3,4,5-F 3 -Phe ( Fig. 5c/d ). These results clearly rule out a cation–pi interaction at position 1767 under tonic or use-dependent conditions as an important factor in drug binding. 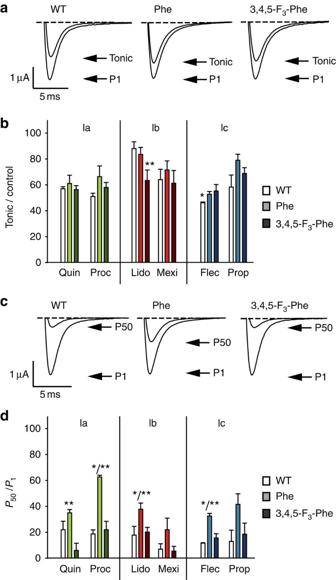Figure 5: Tyr1767 does not form a cation–pi interaction with class I anti-arrhythmics. Tonic (0.2 Hz, (a)) and use-dependent (c) inhibition in the presence of 200 μM mexiletine of WT Nav1.5 (left), or Phe (middle) and 3,4,5-F3-Phe (right) tRNA co-injected with Tyr1767TAG mRNA. Control currents are designated P1, currents remaining after tonic or use-dependent inhibition are designated as tonic and P50, respectively. (b)/(d) Bar diagrams comparing tonic (0.2 Hz) (b) and use-dependent (20 Hz) (d) inhibition of all anti-arrhythmic drugs tested here with WT (white bars); Phe (light coloured bars) or 3,4,5-F3-Phe (dark coloured bars) incorporated at position 1767 (note that WT is shown to account for possible effects of the missing hydroxyl on inhibition by drugs). Data for class Ia drugs Quin and Proc are shown in green, data for class Ib drugs Lido and Mexi are shown in red, data for class Ic drugs Flec and Prop shown in blue. Data shown as mean+s.e.m. (n=3–7). Single and double asterisks indicate significant difference of Phe to WT and Phe to 3,4,5-F3-Phe, respectively (P<0.05; Student'st-test). Flec, flecainide; Lido, lidocaine; Mexi, mexiletine; Proc, procainamide; Prop, propafenone; Quin, quinidine. Figure 5: Tyr1767 does not form a cation–pi interaction with class I anti-arrhythmics. Tonic (0.2 Hz, ( a )) and use-dependent ( c ) inhibition in the presence of 200 μM mexiletine of WT Nav1.5 (left), or Phe (middle) and 3,4,5-F 3 -Phe (right) tRNA co-injected with Tyr1767TAG mRNA. Control currents are designated P 1 , currents remaining after tonic or use-dependent inhibition are designated as tonic and P 50 , respectively. ( b )/( d ) Bar diagrams comparing tonic (0.2 Hz) ( b ) and use-dependent (20 Hz) ( d ) inhibition of all anti-arrhythmic drugs tested here with WT (white bars); Phe (light coloured bars) or 3,4,5-F 3 -Phe (dark coloured bars) incorporated at position 1767 (note that WT is shown to account for possible effects of the missing hydroxyl on inhibition by drugs). Data for class Ia drugs Quin and Proc are shown in green, data for class Ib drugs Lido and Mexi are shown in red, data for class Ic drugs Flec and Prop shown in blue. Data shown as mean+s.e.m. ( n =3–7). Single and double asterisks indicate significant difference of Phe to WT and Phe to 3,4,5-F 3 -Phe, respectively ( P <0.05; Student's t -test). Flec, flecainide; Lido, lidocaine; Mexi, mexiletine; Proc, procainamide; Prop, propafenone; Quin, quinidine. Full size image Early evidence suggested that substitutions at the site equivalent to Phe1760 in neuronal sodium channels can preferentially impact class Ib inhibition, but the molecular basis for this observation has remained unknown [42] . Our results demonstrate that only class Ib anti-arrhythmic drugs form a strong use-dependent cation–pi interaction with Phe1760, whereas the electronegative surface potential at this site makes a less important contribution to inhibition by other class I anti-arrhythmic drugs. We conclude that a strong cation–pi interaction at Phe1760 defines the molecular basis for the inhibition of cardiac sodium channels by class Ib anti-arrhythmic drugs. Not only is this information predictive in defining drug classification, this interaction also represents a significant portion of binding energy, because targeted dispersion of the pi electrons on the face of Phe1760 nearly abolishes the ability of lidocaine or mexiletine to inhibit channels in a use-dependent fashion. We feel these results are insightful because the physicochemical properties of molecular weight, p K a values, partition coefficients, and/or topological polar surface area can explain some of the functional differences between two given anti-arrhythmic drugs [43] , [44] , [45] , [46] , but they fail to be predictive in categorizing the Vaughan-Williams classification scheme ( Table 2 ). Of particular interest are the dramatically different results for the class Ia drug procainamide and the class Ib drug lidocaine, which display very similar physicochemical parameters ( Table 2 ) yet differ in both affinity (lidocaine ≫ procainamide) and reliance on a cation–pi interaction. This is even more surprising because it is the protonated amine of the drug that forms the cation–pi interaction with Phe1760, and procainamide is almost fully protonated at pH 7.4, whereas lidocaine is only about 75% protonated. Why, then, do these drugs differ so fundamentally in their binding mode and affinity? The results with the lidocaine derivatives methyl-4-para-lidocaine, RAD-241, RAD-242 and bupivacaine strongly suggest that both the length and volume of the inhibitor play crucial roles, as more elongated structures with a higher volume can no longer form an energetically significant cation–pi interaction with Phe1760. This is similar to the conclusion of earlier studies that found the affinity of lidocaine derivatives was critically dependent on the length of the linker between the amine and the aromatic groups [46] , [47] . Additionally, longer intermediate chain lengths as well as larger overall sizes will create drugs that can potentially deviate significantly from the planar conformation predicted for lidocaine, mexiletine, RAD-241 and DMAE-B, all of which form energetically significant cation–pi interactions with Phe1760, whereas procainamide, which does not form a cation–pi interaction, displays a kinked backbone structure ( Fig. 2 ), a result consistent with previous work [48] . Similarly, volume generally increases with greater length and size of the drug and although the volume alone cannot be used to classify the anti-arrhythmic drugs used here, we find that only drugs with a volume between 180 and 280 A 3 ( Table 2 ) are capable of forming strong cation–pi interactions. Based on these data, we propose that for a substantial cation–pi interaction with Phe1760 under use-dependent conditions, a compound should have a protonatable amine, an aromatic ring, a molecular volume between 180 and 280 A 3 , and no kinked backbone conformation ( Fig. 2 ; Supplementary Fig. S4 ). In support of this hypothesis, DMAE-B, a compound smaller than procainamide with a planar conformation, forms a cation–pi interaction with Phe1760. Interestingly, the composition of the backbone between the aromatic ring and the amine is not crucial (compare the different linkers of lidocaine, mexiletine and DMAE-B). These data illustrate how subtle manipulations of both interaction partners in drug-receptor interactions can yield valuable information on the defining molecular features of the interaction. Although the importance of Tyr1767 for use-dependent inhibition of Na v 1.5 was recognized very early [22] , [42] , its precise role in this process still remains uncertain. Importantly, robust use-dependent inhibition is only achieved with a tyrosine in position 1767 as other amino-acid substitutions significantly reduce use-dependent inhibition [22] , [41] . Here we show that the introduction of 3,4,5-F 3 -Phe restored inhibition to WT levels, suggesting that an electronegative substituent on the edge of the aromatic (and not the hydrogen-bonding ability of the hydroxyl) at position 1767 is both necessary and sufficient for WT-like inhibition. Simultaneously, these results demonstrate that the negative electrostatic potential on the face of Tyr1767 is not required for inhibition by class I anti-arrhythmic drugs. Our data show that the defining molecular basis for class Ib anti-arrhythmics rely on a strong cation–pi interaction with Phe1760 for use-dependent inhibition; yet, other compounds such as flecainide or ranolazine inhibit the channel with equal or greater affinity without such a requirement, possibly indicating that high affinity inhibition can also be conferred by interactions other than strong cation–pi interactions [12] , [22] , [49] , [50] . This idea is supported by another long-held explanation for these mechanistic differences, which posits that these compounds can interact favourably with distinct conformations within the binding site for local anaesthetics and anti-arrhythmic drugs, thus using an overlapping receptor site but employing distinct molecular interactions. In the case of flecainide, the interaction likely occurs with the open state, whereas lidocaine prefers the inactivated conformation [13] , [51] , [52] , [53] . Our results, therefore, provide a starting point to define a chemical identity to the multiple high-affinity sites within the sodium channel receptor, each representing a valid drug target with different outcomes on heart rhythms. Class Ib drugs show a preference for INa late over INa peak and have the rapid on/off kinetics that are not associated with the pro-arrhythmic prolongation of the action potential seen with other class I drugs, and exhibit little cross reactivity with voltage-gated potassium channels or beta-blocking activity [10] , all features of a safe and salutary anti-arrhythmic compound. Two factors that set the class Ib drugs apart from other class I drugs deserve particular attention: the rapid on/off kinetics, which give rise to the clinically important decrease in the ERP, and the cation–pi interaction with Phe1760. Interestingly, cation–pi interactions are highly dependent on a precise en face orientation [54] . It is thus tempting to speculate that this interaction is a critical factor for the rapid kinetics observed with class Ib drugs: minimal structural changes (see also below) would allow the rapid state-dependent formation or breaking of the interaction. The results of this study are valuable for the informed design of novel therapeutics for the management of cardiac arrhythmia and inhibition of INa late . Furthermore, the approach used here could help with the directed design of novel anti-arrhythmic drugs that specifically target cardiac sodium channels carrying mutations known to cause abnormal channel function in the heart. An interesting aspect of our data is the fact that the observed cation–pi interaction between class Ib anti-arrhythmic drugs and Phe1760 is state-dependent. Specifically, the data clearly argue against a substantial electrostatic contribution of Phe1760 to tonic (or resting) inhibition, but show that a strong cation–pi interaction appears under conditions favouring use-dependent inhibition. This suggests that the DIV S6 helical segment undergoes a conformational change upon repeated depolarization that exposes the previously buried/hidden face of Phe1760 to the permeation pathway and thus allows interaction with drugs that reside in the cavity formed by the S6 segments from all four domains. The idea of a conformational change, possibly a rotation, of DIV S6 during inactivation is supported by previous studies on voltage-gated sodium and potassium channels [55] , [56] , [57] , [58] . Future experiments will help elucidate the nature and extent of this use-dependent conformational change, as this information is crucial for not only understanding therapeutic inhibition, but also voltage-dependent sodium channel function. Molecular Biology and in vivo nonsense suppression The in vivo nonsense suppression methodology was performed with sodium channels as described previously [25] . The Phe1760 and Tyr1767 sites of hNav1.5 complementary DNA were mutated by conventional mutagenesis, and complementary RNA was transcribed from this cDNA (mMessage mMachine, Ambion). Unnatural amino acids (aa) were protected with nitroveratryloxycarbonyl, activated as the cyanomethyl ester, and coupled to the dinucleotide pdCpA (Dharmacon). This aminoacyl dinucleotide was then ligated to a modified transfer RNA from Tetrahymena thermophila . Deprotection of the aminoacylated tRNA-aa was performed by UV irradiation immediately before co-injection with the mRNA for the channel into Stage V–VI Xenopus oocytes. Typically, 20 ng of tRNA-aa and 25 ng of channel cRNA+5.0 ng of β subunit messenger RNA were injected in a 50-nl volume. Injection of oocytes with the Phe1760TAG (or Tyr1767TAG) mRNA alone or in combination with uncoupled tRNA did not produce currents greater than 0.1 μA, ruling out the read-through incorporation of endogenous amino acids or the re-charging of the co-injected tRNA. Computations Gaussian 09/GaussView 5.0 (Wallingford, CT) was used for ab initio gas phase Hartree-Fock 6-31G calculations to generate compound structures and electrostatic potential distribution. Calculated cation–pi interaction energies were modelled with an idealized diffuse cation (in this case ammonium) and a benzene ring. Sequence comparisons for each domain of the cardiac sodium channel (Na V 1.5) were made using ClustalW2 ( http://www.ebi.ac.uk/Tools/msa/clustalw2 ) against the sequence from the S5-pore loop-S6 of the Kv1.2–2.1 paddle chimera (PDB 2R9R ) and displayed in PIR format for use in MODELLER 9v7 (Sali Laboratory), which was used to create the homology model. The specific sodium channel residues were D 252 -E 418 , N 841 -S 942 , N 1336 -N 1474 and G 1661 -S 1776 for DI through DIV, respectively. Domains of the template structure were replaced sequentially with DI, DII, DIII and DIV of the Na V 1.5 sequence, based on homology and using MODELLER. The model was assessed in MODELLER using spatial constraints, steric clashes, Van der Waals and electrostatic contributions. Electrophysiology Voltage-clamped sodium currents were recorded with two microelectrodes using an OC-725C voltage clamp (Warner Instruments) in a standard Ringers solution (in mM): 116 NaCl, 2 KCl, 1 MgCl 2 , 0.5 CaCl 2 , 5 HEPES, pH 7.4. Recordings were performed at 20–22°C, unless noted otherwise. A TC-324B automated temperature controller (Warner Instruments) was used to raise the temperature in the recording chamber when required. Glass microelectrodes had resistances between 0.1 and 1 MΩ and were backfilled with 3 M KCl. The holding potential was −100 mV. Drug application was achieved through an automated perfusion system (Valve Bank 8, AutoMate Scientific). All data=mean±s.e.m. How to cite this article: Pless, S. A. et al . Molecular basis for class Ib anti-arrhythmic inhibition of cardiac sodium channels. Nat. Commun. 2:351 doi: 10.1038/ncomms1351 (2011).